Optofluidic waveguide as a transformation optics device for lightwave bending and manipulation Transformation optics represents a new paradigm for designing light-manipulating devices, such as cloaks and field concentrators, through the engineering of electromagnetic space using materials with spatially variable parameters. Here we analyse liquid flowing in an optofluidic waveguide as a new type of controllable transformation optics medium. We show that a laminar liquid flow in an optofluidic channel exhibits spatially variable dielectric properties that support novel wave-focussing and interference phenomena, which are distinctively different from the discrete diffraction observed in solid waveguide arrays. Our work provides new insight into the unique optical properties of optofluidic waveguides and their potential applications. Transformation optics [1] is currently an area of intense investigation [2] , [3] , [4] , [5] , [6] , representing a new paradigm for the manipulation of light by using materials that exhibit spatially variable distributions of permittivity and permeability to alter the electromagnetic space. Initially, transformation optics research was focussed on exploiting both the magnetic and electric responses of the medium. However, a number of systems with spatially variant permittivity and fixed unitary permeability have been identified recently, offering new and exciting opportunities for controlling and manipulating light. Applications include imperfect dielectric cloaking [7] , carpet cloaking [8] , [9] , [10] and Luneberg lenses [11] . In addition, the transformation optics approach has been used to improve the optical properties of conventional refractive and gradient-index (GRIN) optical imaging devices [12] , [13] . To date, experimental transformation optics research has exploited only solid dielectric materials, as artificial metamaterials require complicated fabrication processes [8] , [14] . Optofluidic research draws its strengths from both fluid dynamics and optics. It has inspired the creation of a variety of innovative devices [15] , [16] , [17] , [18] , in particular, devices controlled by flow rates and liquid compositions [19] , [20] , [21] , [22] , [23] . Here we show the first observation of the distinctive phenomena of chirped focussing of light and interference in an optofluidic waveguide underpinned by a unique bidirectional refractive index gradient profile in a flow channel. This effect depends on the characteristics of the waveguide, the liquid composition and the flow rate. We argue that our observations represent a demonstration of a controllable transformation optics device based on a liquid medium. 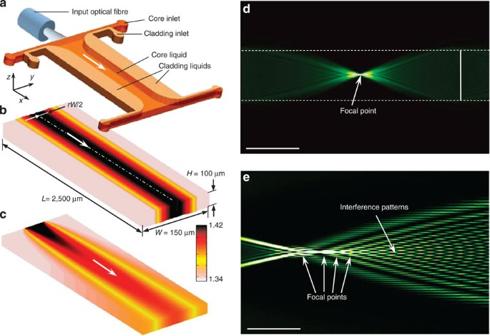Figure 1: Design of light focussing and interference in an optofluidic waveguide. (a) Schematic illustration of the optofluidic waveguide with three laminar flows in the microchannel (the surrounding PDMS structures are not shown). The white arrow represents the flow direction. (b) GRIN profile of the microchannel in the transverse direction used to achieve light focussing. (c) Bidirectional GRIN profile used to achieve light interference. The intensity scale shows the refractive index distribution. (d) Simulated light propagation in the waveguide for the index profile shown in (b), wheren(0)=1.432,nc=1.332. Light is bent and periodically focussed in the optofluidic waveguide. The horizontal dashed lines represent the boundaries between the waveguide core and claddings. The vertical solid line represents the wavefront. (e) Simulated light propagation in the waveguide with the index profile shown in (c), wherer=1/3 andQclad=0.5 μl min−1. Light interference is clearly shown in the optofluidic waveguide. For (d) and (e), scale bar equals 100 μm and the vertical direction is magnified by two. Light bending in the optofluidic waveguide Figure 1a shows a typical design of the optofluidic waveguide, which consists of three flow streams. The central flow stream is injected with a liquid of relatively high-refractive index compared with the side-flow streams. The details of the fabrication processes and experimental conditions are discussed in the Methods. In such a waveguide, we investigated two different light-propagation phenomena and compared our results by using finite-difference time-domain calculations. Figure 1: Design of light focussing and interference in an optofluidic waveguide. ( a ) Schematic illustration of the optofluidic waveguide with three laminar flows in the microchannel (the surrounding PDMS structures are not shown). The white arrow represents the flow direction. ( b ) GRIN profile of the microchannel in the transverse direction used to achieve light focussing. ( c ) Bidirectional GRIN profile used to achieve light interference. The intensity scale shows the refractive index distribution. ( d ) Simulated light propagation in the waveguide for the index profile shown in ( b ), where n (0)=1.432, n c =1.332. Light is bent and periodically focussed in the optofluidic waveguide. The horizontal dashed lines represent the boundaries between the waveguide core and claddings. The vertical solid line represents the wavefront. ( e ) Simulated light propagation in the waveguide with the index profile shown in ( c ), where r =1/3 and Q clad =0.5 μl min −1 . Light interference is clearly shown in the optofluidic waveguide. For ( d ) and ( e ), scale bar equals 100 μm and the vertical direction is magnified by two. Full size image First, we investigated the waveguide regimes leading to the light-focussing phenomenon in the waveguide, which requires a gradient refractive index profile in the transverse direction, as shown in Figure 1b . Such a profile can be achieved by tuning the flow rates, as will be discussed in the next section. The results of simulations ( Fig. 1c ) show the curved light-ray trajectories converging to a focus at a distance of 300 μm from the core inlet. To achieve a longer focal distance, a milder GRIN profile is required. Second, we investigated the waveguide regimes leading to light interference in the waveguide. To observe a strong interference effect with analogous discrete diffraction, a bidirectional GRIN profile (in both the transverse and propagation directions) is needed, as shown in Figure 1d,e . Such a profile can be achieved by tuning the flow rates, as will be discussed in the next section. An analytical explanation of light propagation in a bidirectional GRIN waveguide is presented in the Methods. Control of the continuous GRIN profile Optofluidic waveguides provide an opportunity to tune the spatial distribution of the refractive index in the microchannel. In our system, a core liquid stream (ethylene glycol, n core =1.432) and two identical cladding liquid streams (de-ionized water, n clad =1.332) were pumped into the microchannel through the inlets. As the core flow stream has a refractive index higher than that of the cladding flow streams and the poly-dimethyl siloxane (PDMS) [16] , [18] of the supporting substrate structure, the light can be confined in both the transverse and vertical directions (that is, y and z directions). The refractive index profile in the optofluidic waveguide is determined by the Péclet number (Pe) of the flow, which is a dimensionless parameter defined by the ratio of the advection rate to the diffusion rate between the liquids in the optofluidic waveguide. At high Pe, advection dominates, but diffusion becomes dominant at low Pe, when an inhomogeneous optical medium with gradient parameters can be formed. Importantly, the Pe can be tuned by varying the core size of the fluid channel and the flow rates. We argue that the optofluidic waveguides of different construction but exhibiting Pe similar to those reported here, that is, less than 0.001, will show similar wave propagation and interference effects. More details are given in the Methods. A bidirectional GRIN-like profile can be achieved at a relatively slow flow rate, because diffusion causes the core/cladding interface to smear downstream (see Fig. 2a for a cladding flow rate Q clad =0.5 μl min −1 and r =1/3; here, r is defined as the position of the core/cladding interface with respect to the half width of the microchannel). Such an effect is better presented with reference to the cross-sectional refractive index profiles along the flow streams in the x direction ( Fig. 2b ). At x =0, the flow stream clearly shows a step-index profile because the core liquid and the cladding liquids begin to come into contact. At x = L /2, the profile becomes smoother such that the sharp core/cladding flow stream interface disappears. The peak value of the refractive index at the core centre is lowered, but a GRIN profile can be obtained in the transverse direction (that is, the y direction). At x = L , the GRIN profile is further relaxed. This continuously varying profile differs from that of the traditional solid material GRIN profile with a transverse GRIN component that is homogeneous in the propagation direction. 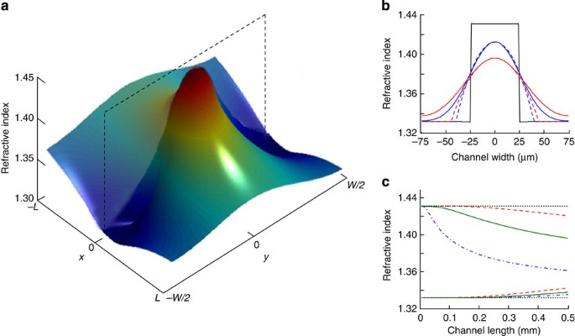Figure 2: Control of the diffusion-induced bidirectional GRIN profile. (a) Calculated refractive index profile forr=1/3 as a result of diffusion at a low flow rate ofQclad=0.5 μl min−1. The dashed black line indicates thex=0 line. (b) Cross-sectional refractive index profiles of (a) atx=0 (solid black),L/2 (solid blue) andL(solid red), where the dashed blue and red lines represent the fitted power law curves. (c) Calculated refractive indexncoreat the core central line (upper lines) andncladat the core/cladding interface (lower lines) withQclad=0.5 μl min−1, withr=1/2 (dashed red),r=1/3 (solid green) andr=1/6 (dash-dotted blue). The dotted black lines represent the high-flow-rate-induced step-index profile in (b). Figure 2: Control of the diffusion-induced bidirectional GRIN profile. ( a ) Calculated refractive index profile for r =1/3 as a result of diffusion at a low flow rate of Q clad =0.5 μl min −1 . The dashed black line indicates the x =0 line. ( b ) Cross-sectional refractive index profiles of ( a ) at x =0 (solid black), L /2 (solid blue) and L (solid red), where the dashed blue and red lines represent the fitted power law curves. ( c ) Calculated refractive index n core at the core central line (upper lines) and n clad at the core/cladding interface (lower lines) with Q clad =0.5 μl min −1 , with r =1/2 (dashed red), r =1/3 (solid green) and r =1/6 (dash-dotted blue). The dotted black lines represent the high-flow-rate-induced step-index profile in ( b ). Full size image For further comparison, the calculated profiles are fitted to the power-law profile of the waveguide, which is the cross-sectional index profile of the waveguide (detailed discussions are given in the Methods). The curves of α =2 correspond to the refractive index profiles of the typical GRIN lenses and fibres, where light undergoes a well-known self-focussing effect [24] , [25] , [26] . Figure 2c shows that the calculated profile fits well to the α =2 profile in the core region, but deviates significantly in the cladding region. To reflect the GRIN in the longitudinal direction (that is, the x direction), the refractive index n core at the core centre y =0 and n clad in the original core/cladding interface y = rW / 2 are plotted in Figure 1e as functions of the channel length. For comparison, the step-index profile at 50 μl min −1 (Pe=0.07), and another two cases of r =1/6 (Pe=0.0005) and r =½ (Pe=0.001) at 0.5 μl min −1 , are also presented. Both n core and n clad vary with the channel length L and the core width r . This observation shows that the GRIN in the longitudinal direction can be tuned by simply adjusting the flow rate ratio of the core fluid and the cladding fluid. Comparison of the experimental results and simulations The experimentally observed light focussing and interference are compared with the simulations. 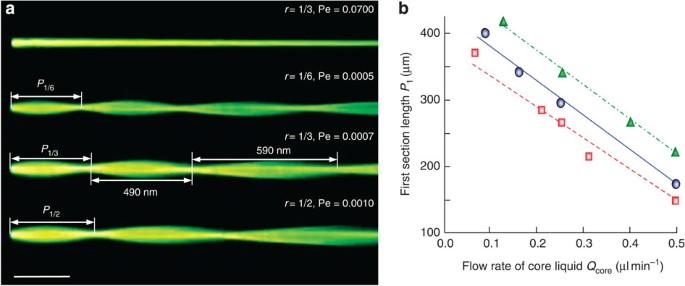Figure 3: Focussing of light in the optofluidic waveguides. (a) Observed light propagation under different flow conditions. At a high flow rate ofQclad=50 μl min−1, the light is confined in the core due to the step-index distribution. AtQclad=0.5 μl min−1, the diffusion-induced gradient of the refractive index causes the light to repeatedly merge. With increasingr, the length of the first section becomes larger, for example,P1/6=270 μm,P1/3=300 μm andP1/2=340 μm. The focussing period also increases, for example, the first period forP1/3is 300 μm, the second is extended to 490 μm and the third is 590 μm. (Scale bar equals 300 μm). (b) The first section lengths as a function of the flow rate of the core fluid atr=1/6 (square),r=1/3 (circle) andr=1/2 (triangle), showing an approximately linearly decreasing relationship over aQcladrange of 0.1–1.0 μl min−1. Figure 3a shows light propagation in the optofluidic waveguides under different fluidic conditions. When driven at a high-flow rate of Q clad =50 μl min −1 (Pe=0.07), the light propagates in a straight line and shows no focussing effect, which is expected because the optofluidic waveguide resembles a step-index waveguide. In contrast, at a low flow rate of Q clad =0.5 μl min −1 , the light exhibits curved-ray trajectories and converges repeatedly for different core widths, r =1/6, 1/3 and 1/2 (Pe=0.0005, 0.0007 and 0.001, respectively). The length of the first section increases with the core width and decreases almost linearly with the flow rate of the core fluid ( Fig. 3b ). However, when examining the light propagation pattern in detail, it is found that the self-focussing period is chirped such that the focussing period increases. For instance, the first period for P 1/3 is 300 μm, the second is extended to 490 μm, and the third is 590 μm, as shown in Figure 3a , owing to the diminishing bidirectional gradient contrast downstream as a result of diffusion. Such chirping is distinct from the focussing seen for the fixed period of conventional GRIN waveguides. Figure 3: Focussing of light in the optofluidic waveguides. ( a ) Observed light propagation under different flow conditions. At a high flow rate of Q clad =50 μl min −1 , the light is confined in the core due to the step-index distribution. At Q clad =0.5 μl min −1 , the diffusion-induced gradient of the refractive index causes the light to repeatedly merge. With increasing r , the length of the first section becomes larger, for example, P 1/6 =270 μm, P 1/3 =300 μm and P 1/2 =340 μm. The focussing period also increases, for example, the first period for P 1/3 is 300 μm, the second is extended to 490 μm and the third is 590 μm. (Scale bar equals 300 μm). ( b ) The first section lengths as a function of the flow rate of the core fluid at r =1/6 (square), r =1/3 (circle) and r =1/2 (triangle), showing an approximately linearly decreasing relationship over a Q clad range of 0.1–1.0 μl min −1 . Full size image To achieve light interference in the optofluidic waveguide (Pe=0.0007), the parameters are set to r =1/3 and Q clad =0.5 μl min −1 . 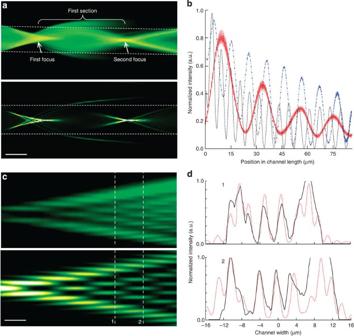Figure 4: Interference patterns in the optofluidic waveguide. (a) Zoomed-in views of the first section from the experimental observation (top) and from the simulation using the finite-difference time-domain method (bottom) forQclad=0.5 μl min−1,r=1/3. In (a), the vertical direction is magnified by two and the dashed lines indicate the region of core liquid without diffusion. A rough matching can be observed between the measured ray trajectories and the simulated field distribution patterns. (Scale bar equals 100 μm). (b) Intensity profiles along the central line in the first section (solid red), second section (dash-dotted blue) and third section (dotted black), respectively, showing that the light is not evenly distributed in the off-focal regions, which suggests the presence of interference patterns in the optofluidic waveguides. (c) Observed (top) and simulated (bottom) interference patterns in the optofluidic waveguide. (Scale bar equals 15 μm). (d) Comparison of the intensity profiles along the monitoring lines 1 and 2 in (c) for the measured (solid black) and simulated (dotted red) patterns. The positions and relative intensities of the bright spots show a rough agreement. The discrepancy is mainly attributed to the imperfection of the flow control (a.u. stands for arbitrary units). The optical micrograph of light distribution near the first section is shown in Figure 4a . Beyond the first focal point, most rays bend in quickly to the second focal point, but some fan out and converge slowly, forming fin-like patterns. For comparison, corroborating simulated light propagation traces are also shown in Figure 4a . The intensity distribution along the central line of the optofluidic waveguide is plotted in Figure 4b . It is obvious that the intensity in any focal section exhibits a large variation resulting from the interference effect. A close-up of the region just beyond the focal point shows the interference patterns, in which regular bright spots appear within an open angle of 12° ( Fig. 4c ). The patterns look very similar to the simulated results presented in Figure 4c , although some bright spots in the upper left corner of the measured patterns are blurry, owing to the scattering of dye molecules and imperfect fluidic control. A detailed comparison of the intensity profiles along two monitoring lines is shown in Figure 4d . An overall agreement in terms of the positions and relative intensities of the bright spots was obtained. The interference effect originates from the bidirectional refractive index gradient profile of the optofluidic waveguides; rays entering from different positions on the input side follow different trajectories and thus exhibit variable phase changes. Detailed theoretical explanations describing the amplitude and phase distribution of light in a two-dimensional inhomogeneous optical medium [25] , [26] are presented in the Methods. The interference effect in the optofluidic waveguides may appear similar to the well-studied discrete diffraction phenomenon [27] . Figure 4: Interference patterns in the optofluidic waveguide. ( a ) Zoomed-in views of the first section from the experimental observation (top) and from the simulation using the finite-difference time-domain method (bottom) for Q clad =0.5 μl min −1 , r =1/3. In ( a ), the vertical direction is magnified by two and the dashed lines indicate the region of core liquid without diffusion. A rough matching can be observed between the measured ray trajectories and the simulated field distribution patterns. (Scale bar equals 100 μm). ( b ) Intensity profiles along the central line in the first section (solid red), second section (dash-dotted blue) and third section (dotted black), respectively, showing that the light is not evenly distributed in the off-focal regions, which suggests the presence of interference patterns in the optofluidic waveguides. ( c ) Observed (top) and simulated (bottom) interference patterns in the optofluidic waveguide. (Scale bar equals 15 μm). ( d ) Comparison of the intensity profiles along the monitoring lines 1 and 2 in (c) for the measured (solid black) and simulated (dotted red) patterns. The positions and relative intensities of the bright spots show a rough agreement. The discrepancy is mainly attributed to the imperfection of the flow control (a.u. stands for arbitrary units). Full size image We have demonstrated chirped focussing and light interference that can be seen only in multi-mode optofluidic waveguides and are not possible in a single-mode waveguiding structure (see Supplementary Movie 1 ). This work focussed on low-flow-rate optofluidic waveguides, in which a continuous variation of the refractive index occurs. The physics governing light propagation effects in such waveguides differs from that of conventional liquid–liquid waveguides. In low-flow-rate optofluidic waveguides, diffusion has a greater role in creating an inhomogeneous optical medium that allows the new complex phenomena of self-focussing and interference. Indeed, conventional high-flow-rate liquid–liquid waveguides are usually operated at high Pe, often 10–100 times larger than those studied here [16] , [18] . As a result, in the high-flow-rate waveguides, diffusion has a limited role, and the waveguides act as step-index optical waveguides, as shown in Supplementary Figure S1 . In the study reported here, the optofluidic waveguides operate at a Pe of less than 0.001, leading to the creation of an inhomogeneous optical medium in which variations in the refractive index occur on a scale that is comparable to, but larger than, the wavelength of light (see Supplementary Fig. S2 ). When light propagates in a waveguide with a GRIN profile, loss through leakage at the channel/liquid interface occurs. This energy loss has been estimated by the intensity of fluorescent emission and found to be approximately 3 dB in a 2,500-μm microchannel for the case of extreme diffusion ( r =1/6, Q =1 μl min −1 ). This leakage loss can be reduced by replacing the de-ionized water with an ethylene glycol–water mixture, which has a higher refractive index than PDMS [16] , [18] . However, this substitution will reduce the index contrast of the two liquid flow streams and will limit the device tunability. The convection–diffusion process is unique to miscible liquids and is not observed in solid materials. The low-flow-rate optofluidic waveguide system is a new material system with controllable, spatially variable dielectric parameters, and is a good candidate for designing transformation optics experiments with GRIN profiles controllable by the variation of flow rates. The diffraction and interference of light in the optofluidic waveguides occur in a very different manner than in a solid waveguide array; the optofluidic waveguide is a system with spatially variable and actively controllable dielectric characteristics, which can be tuned by changing the fluid flow rate. Here, discrete diffraction patterns arise from the self-focussing effect due to the transverse index-gradient profiles. In conclusion, two distinctive phenomena of the optofluidic waveguides have been demonstrated and controlled: chirped focussing and light interference. These phenomena rely on the continuous GRIN profile, which is controlled by microfluidic manipulation. With inherent real-time tunability and reconfigurability, such waveguides may be the versatile platforms for many scientific studies, particularly in dynamically controlled transformation optics systems. These new phenomena have potential applications in the GRIN-like optical elements for optical modulation and signal routing, which can be achieved by manipulating the light distribution via the control of liquid flow rates. In addition, the interference patterns may be applied to nanoparticle bunching, sorting and dynamic assembling using the optical gradient force [28] , which depends on the sizes and refractive indices of the particulates. Simulating the optofluidic waveguide GRIN profile An optofluidic waveguide is predominantly governed by the diffusion and convection processes between the core fluid and the cladding fluid. The convective–diffusive transport can be expressed as [29] where C is the concentration, D is the diffusion coefficient, U is the velocity and t is the time. The first term on the right side corresponds to normal diffusion and the second term describes convection. For a steady-state flow, the concentration does not vary with time, and thus, the term on the left side Under some assumptions and conditions, the numerical model can be simplified to two dimensions. The concentration distribution for the fully developed, steady-state flow in the microchannel can be expressed as [30] where and are the normalized coordinates and is the normalized concentration. The boundary conditions include c ′| x ′=0, 0≤ y ′< r =1, c ′| x ′=0, y ′= r = r and c ′| x ′=0, r ≤ y ′≤1 =0 for the initial state, for the full mixing state at the outlet and at the PDMS wall, respectively. Here we chose an xyz coordinate system and let the flow direction be along x , the channel width along y and the channel height along z ( Fig. 1a ). Pe = UW / D is the Péclet number, is the average velocity, Q core is the flow rate of the core fluid, Q clad is the flow rate of each of the cladding fluids, W and H are the width and height of the microchannel, respectively. The variable r is the normalized initial boundary ratio between the core and cladding fluids and can be derived from [31] where and μ 1 and μ 2 are the viscosities of the two fluids, respectively. In this work, the geometry of the microchannel and the diffusion coefficients of the selected liquids are fixed, and thus, the flow rates of the core and cladding fluids govern the final concentrations. At a high flow rate, the Pe is relatively large. Subsequently, the concentration distribution is approximately constant within a limited waveguide length, as occurs with the step-index optofluidic waveguide previously described. However, when the flow rate is reduced, concentration gradients exist in both the longitudinal and transverse directions (that is, x and y directions). As a result, a refractive index gradient is created in the microchannel. The index profile n ( x ′, y ′) can be derived from the concentration profile of the two liquid components: Similarly, index gradients exist in both the longitudinal and transverse directions, presenting a difference from conventional solid GRIN waveguides, which have an index gradient only in the transverse direction. Fitting of the power-law profile of the waveguide For comparison, the calculated profiles in Figure 1b were fitted to the power-law profile of the waveguide, as given by Snyder and Love [32] where n ( x , y ) is the refractive index at the point ( x , y ), n core ( x , 0) is the refractive index at the core centre ( x , 0), , n clad is the refractive index of the homogeneous cladding layer, ρ is the normalized core width as given by and α is the parameter that defines the shape of the profile. Equation (4) becomes a step-index profile in the limit of α→+∞. It is well known that α =2 yields a sine function for the ray trajectories and thus, periodic focussing for all of the rays. In Figure 1d , the refractive index profile at x =0 can be fitted exactly to α=+∞ and those at x = L /2 and x = L are approximately fitted to α =2. In the latter two fittings, the fitted curves match closely with the diffusion-induced gradient profiles within the original core region, but deviate significantly outside of this area. The fitted curves have sharp stops at certain locations, but the gradient profiles exhibit smooth tails. It seems that the rays that travel within the original core region still follow periodic trajectories, whereas the other rays do not. However, as the gradient profile varies in the flow direction, the ray trajectories become more complicated. Light propagation in a bidirectional GRIN waveguide The theoretical model of light propagation in an inhomogeneous layer is shown in Supplementary Figure S3 . Variations in the refractive index can be obtained by calculating the first-order partial derivatives of the normalized concentration c ′ in equation (2), with respect to the normalized coordinates x ′ and y ′, which can be written as Both equations reduce to when Pe→0; thus, is comparable to and the gradient in the x direction cannot be ignored when the flow rate is low. As the wave function of an arbitrary incoming light ray can be decomposed into a series of monochromatic plane waves using a Fourier transformation, the propagation of a monochromatic plane wave ψ ( x , y ) in a two-dimensional layer must be considered. For simplicity, ψ ( x , y )= ψ ( x ) ψ ( y ). From the wave equation [26] , where k is the wave vector, A 1 , A 2 , and represent the transmission and reflection coefficients, respectively. On the basis of equation (6), the amplitude and phase of the light can be calculated. Ray tracing can also be satisfied by the relationship where y 1 is the position of the ray (see Supplementary Fig. S3 ). With these analytical equations, the propagation of light in the optofluidic waveguide can be investigated. For verification and comparison, the well-known graded-index fibre is studied as well. For incident light travelling along the x direction, we have θ 0 =0, and The initial conditions are n core (0)=1.432 and n clad =1.332 for the unidirectional graded-index fibre, and n core (0, 0)=1.432 and n clad (0, y ′)=1.332 for the bidirectional GRIN optofluidic waveguide. On the basis of equation (8), ray tracing is conducted as shown in Supplementary Figure S4 . In a graded-index fibre, the incoming rays entering from different transverse locations follow different trajectories but converge to a single focal point, because the phases of the different rays are almost the same at the focal point, exhibiting the well-known self-focussing effect. Beyond this focal point, the rays continue at different open angles and follow different trajectories. The rays are well separated from each other and thus, do not intersect, causing no obvious interference. However, in the optofluidic waveguide, the incoming rays converge to different locations, because the waveguide has a rapid change of refractive index near the initial core/cladding interface, but a smooth change close to the core centre (refer to the slope of the refractive index curves in Fig. 2a ). As a result, the rays at the centre require a long distance for convergence (that is, have a longer period), whereas those in the outside regions have a shorter period (see Supplementary Fig. S4b ). Therefore, the incoming rays converge to different locations, resulting in multiple focal points. For this reason, the rays have intersecting trajectories and thus interfere with each other to create bright and dark spots, forming the interference patterns. On the basis of equation (7), the intensity distributions of the light are shown in Figure 1 . For the graded-index fibre, the self-focussing effect is well reproduced in Figure 1d , which verifies the effectiveness of the theoretical model. For the optofluidic waveguide, the intensity distribution indeed exhibits multiple focal points and strong interference patterns, as predicted by the above ray tracing discussion. The interference patterns agree well with the experimental observation and the simulated results obtained using the finite-difference time-domain method. These data confirm that the theoretical explanation can describe the main features of the optofluidic waveguide. Fabrication processes and experimental setup The microchannel system was fabricated using soft-lithography processes. First, photoresist-on-silicon masters of the microchannels were prepared in a cleanroom by photolithography (Micro-Chem, SU-8) using transparent glass masks (CAD/Art Services Inc., Poway, CA, USA). Then, the microchannels were molded using PDMS and sealed against flat PDMS slabs after plasma oxidation [33] . The microchannel has an index of n PDMS =1.405 and dimensions of L =2,500μm, W =150μm and H =100 μm. The core liquid is ethylene glycol ( n core =1.432) and the cladding liquid is de-ionized water ( n clad =1.332). As the refractive index of the core fluid is higher than that of the cladding fluid and the PDMS, the light can be confined in both the horizontal and vertical directions. An argon ion laser (488 nm, Melles Griot, 35-LAP-431-230) was coupled to an optical fibre (cladding diameter: 125 μm, core diameter: 9 μm) and delivered to the optofluidic waveguide. The image was captured using an inverted optical microscope (TS 100 Eclipse, Nikon) through a charge-coupled device camera (DS-Fil, Nikon). The liquids were injected using syringe pumps (Genie, Kent Scientific Corporation, CT, USA). For fluorescence imaging, rhodamine 6G with a concentration of 1×10 −7 mol l −1 (excitation: 488 nm, emission: 550–590 nm) was added. As of the use of rhodamine 6G, the ray trajectories in the optofluidic waveguide were visible. The miscibility of the ethylene glycol and de-ionized water ensures a diffusion of the two liquids (and the dye) in the laminar flow regime and leads to a change in the refractive index distribution. The diffusion coefficient for dilute aqueous solutions of ethylene glycol is 1.16×10 −5 cm 2 s −1 (ref. 34 ). How to cite this article: Yang, Y. et al . Optofluidic waveguide as a transformation optics device for lightwave bending and manipulation. Nat. Commun. 3:651 doi: 10.1038/ncomms1662 (2012).